Rag GTPases are cardioprotective by regulating lysosomal function The Rag family proteins are Ras-like small GTPases that have a critical role in amino-acid-stimulated mTORC1 activation by recruiting mTORC1 to lysosome. Despite progress in the mechanistic understanding of Rag GTPases in mTORC1 activation, little is known about the physiological function of Rag GTPases in vivo. Here we show that loss of RagA and RagB (RagA/B) in cardiomyocytes results in hypertrophic cardiomyopathy and phenocopies lysosomal storage diseases, although mTORC1 activity is not substantially impaired in vivo . We demonstrate that despite upregulation of lysosomal protein expression by constitutive activation of the transcription factor EB (TFEB) in RagA/B knockout mouse embryonic fibroblasts, lysosomal acidification is compromised owing to decreased v-ATPase level in the lysosome fraction. Our study uncovers RagA/B GTPases as key regulators of lysosomal function and cardiac protection. Rag family proteins (Rag A, B, C and D) are a unique subgroup of the Ras GTPase superfamily. Unlike other Ras family proteins, Rag GTPases are significantly larger and form heterodimers. For example, RagA or RagB forms a stable complex with RagC or RagD, with the possibility of forming four distinct complexes [1] . RagA was initially identified as a functional homologue of the yeast Gtr1 that also forms a heterodimer with Gtr2 (homologous to RagC and RagD). Genetic studies revealed that Gtr1/Gtr2 is involved in various cellular processes such as nuclear transport, microautophagy and intracellular trafficking [2] , [3] , [4] . Our group and Sabatini’s laboratory discovered that the Rag GTPases have an essential role in amino-acid-mediated mechanistic target of rapamycin complex1 (mTORC1) activation [5] , [6] . The heterodimer formation of Rag GTPases is critical for mTORC1 activation, but RagA/B appears to be more important than RagC/D in mTORC1 activation. Thus, overexpression of the constitutively active form (GTP-bound mutant) of RagA (or B), regardless of the nucleotide status of RagC (or D), can activate mTORC1 even in the absence of amino acids [5] , [6] . It has been reported that amino acids can stimulate RagA/B and RagC/D to bind GTP and GDP, respectively [6] , therefore leading to mTORC1 activation. However, a recent study showed that the binding of Rag GTPases to mTORC1 is regulated by amino acids without altering GTP charging of the Rag GTPase heterodimer, suggesting that additional mechanisms may be involved in amino-acid-induced mTORC1 activation [7] . Rag GTPases are anchored on the surface of lysosomes by a protein complex called Ragulator in close proximity to Rheb [8] . The active Rag heterodimeric complex (RagA/B GTP-bound and RagC/D GDP-bound) binds directly to Raptor, a subunit of the mTORC1 complex, thereby recruiting the kinase complex to lysosome. At the lysosome, the mTORC1 is activated by Rheb that mediates growth factor signals by acting downstream of the TSC1/TSC2 GTPase activating protein (GAP) [9] , [10] . The Ragulator also functions as a guanidine exchange factor for RagA/B and connects the v-ATPase (vacuolar H + -adenosine triphosphatase) to the Rag GTPases for mTORC1 activation by amino acids [11] , [12] . Therefore, Rag GTPases mediate amino-acid signals by recruiting the mTORC1 complex to lysosome. Lysosomes are cellular organelles that hydrolyse metabolites and cellular wastes to maintain cellular homeostasis or recycling of nutrients. Lysosomal dysfunction caused by genetic mutations in lysosomal proteins causes lysosomal storage diseases (LSDs). Thus, LSDs are associated with abnormal accumulation of metabolites, and the major affected organs are the metabolic centres of the body such as liver, skeletal muscle and heart [13] , [14] . Rag GTPases-mTORC1 signalling regulates lysosomal biogenesis via transcription factor EB (TFEB), which promotes lysosomal protein expression [15] , [16] , [17] . Rag GTPases and mTORC1 regulate TFEB by direct binding and phosphorylation, respectively. Intriguingly, overexpression of TFEB can facilitate autophagy flux and ameliorate LSDs in vitro and in vivo [18] , [19] , [20] . Therefore, it is conceivable that the downregulation of Rag GTPases-mTORC1 signalling may facilitate lysosome function due to TFEB activation. In this study, we investigated the physiological function of Rag GTPases using conditional knockout (KO) mice. We show that loss of RagA/B in cardiomyocytes causes cardiac hypertrophy and phenocopies LSDs. Moreover, we demonstrate that despite constitutive activation of TFEB, the lysosomal expression of v-ATPase is decreased in RagA/B KO cells, resulting in compromised lysosomal acidification and dysfunction. Our study provides new insights into the critical physiological functions of RagA/B in heart and defines a novel role of Rag GTPases in lysosomal function by regulating lysosomal v-ATPase expression. Loss of RagA and RagB in heart causes cardiac hypertrophy Formation of heterodimer is essential for Rag GTPase function and stability. Therefore, we reasoned that deletion of both RagA and RagB , which are highly homologous and functionally redundant, should be sufficient to inactivate the Rag GTPases. To investigate the physiological role of Rag GTPases in specific tissues, we generated RagA and RagB double conditional KO mice using the Cre- loxP system ( Supplementary Fig. 1A ). Since Rag GTPases regulate amino-acid-mediated mTORC1 activation [5] , [6] , and mTORC1 signalling has a critical role in the muscle tissues [21] , [22] , [23] , [24] , we used a transgenic mouse model that expresses Cre recombinases under the control of muscle creatine kinase promoter (Mck-Cre) to delete the floxed alleles in skeletal and cardiac muscle tissues [25] . In the course of generating Mck-Cre /+ ;RagA fl/fl ;RagB fl/fl (hereinafter RagA/B cKO), we first confirmed the Cre-mediated deletion of floxed alleles in RagA fl/fl or RagB fl/fl mice using genomic DNA (gDNA) PCR analyses ( Supplementary Fig. 1B ). Although the recombination of floxed alleles by Cre was detected in skeletal muscles, we were surprised that the RagA protein levels were not significantly reduced in the RagA/B cKO muscles ( Supplementary Fig. 2B ). Moreover, we did not find any noticeable pathological phenotypes in skeletal muscles of RagA/B cKO mice ( Supplementary Fig. 2 ). Based on these observations, we speculate that the lack of phenotype in the skeletal muscles of RagA/B cKO mice is probably because of both the incomplete deletion (<100%) of the floxed alleles by the Cre recombinase and the presence of multiple nuclei (some with RagA/B deletion and some with no RagA/B deletion) in skeletal muscle fibres. Therefore muscle fibres still have some myofibre nuclei in which RagA and RagB are not deleted. On the other hand, loss of RagA and RagB in cardiomyocytes caused severe cardiac hypertrophy ( Figs 1 and 2 ). Unlike the skeletal muscle, the RagA protein levels were significantly reduced in the heart tissues of RagA/B cKO mice ( Fig. 1a ). Because the anti-RagA antibody could also weakly detect RagB, we found that RagB protein was detected in the control heart tissues, but not in the RagA/B cKO hearts (arrowhead in Fig. 1a ), showing that both RagA and RagB floxed alleles were efficiently deleted by Cre in the heart. 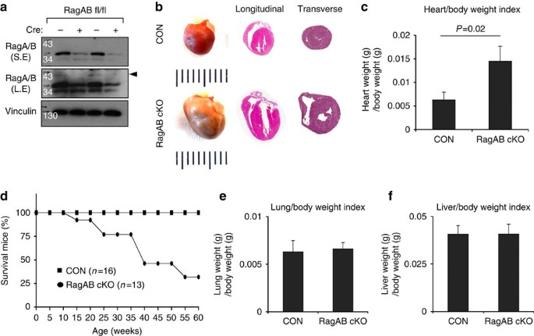Figure 1: Loss ofRagAandRagBcauses cardiomegaly and premature death. (a) RagA and RagB protein levels are decreased in RagA/B cKO hearts. Heart tissue lysates were prepared from control or RagA/B cKO mice and analysed by immunoblotting. S.E., short exposure; L.E., long exposure. (b) Representative images of whole-mount hearts (4 months old), and haematoxylin and eosin-stained longitudinal and transverse sections of the hearts from 4-month and 1-year-old mice, respectively. Ruler represents 1 mm per interval. (c) Heart/body weight index. Heart weight was divided by body weight. Values represent the mean±s.d. of data (n=8 per group).P=0.02, Wilcoxon rank sum test. (d) Survival curve of control and RagA/B cKO mice.P<0.00001, Mantel–Cox (log-rank) test. (e) Lung/body weight index. Lung weight was divided by body weight of the mouse. Values represent the mean±s.d. of data (n=8 per group). (f) Liver/body weight index. Liver weight was divided by body weight of the mouse. Values represent the mean±s.d. of data (n=8 per group). CON, control. Figure 1: Loss of RagA and RagB causes cardiomegaly and premature death. ( a ) RagA and RagB protein levels are decreased in RagA/B cKO hearts. Heart tissue lysates were prepared from control or RagA/B cKO mice and analysed by immunoblotting. S.E., short exposure; L.E., long exposure. ( b ) Representative images of whole-mount hearts (4 months old), and haematoxylin and eosin-stained longitudinal and transverse sections of the hearts from 4-month and 1-year-old mice, respectively. Ruler represents 1 mm per interval. ( c ) Heart/body weight index. Heart weight was divided by body weight. Values represent the mean±s.d. of data ( n =8 per group). P =0.02, Wilcoxon rank sum test. ( d ) Survival curve of control and RagA/B cKO mice. P <0.00001, Mantel–Cox (log-rank) test. ( e ) Lung/body weight index. Lung weight was divided by body weight of the mouse. Values represent the mean±s.d. of data ( n =8 per group). ( f ) Liver/body weight index. Liver weight was divided by body weight of the mouse. Values represent the mean±s.d. of data ( n =8 per group). CON, control. 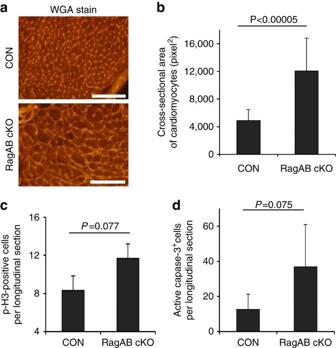Figure 2: Cardiac hypertrophy in RagA/B cKO mice. (a) Images of wheat germ agglutinin (WGA)-stained heart tissues. Representative images from control and RagA/B cKO tissues are shown. Scale bars, 100 μm. (b) Cross-sectional area of cardiomyocytes. The area of cardiomyocytes fromawas measured using the ImageJ software. Values represent the mean±s.d. of data (n=15 per group). (c) Quantification of cell proliferation in heart tissues. Longitudinal sections of whole mount of hearts were stained with phsopho-Histone3 (p-H3) antibody to detect proliferating cardiomyocytes. The p-H3-positive cells in a whole longitudinal tissue section were counted. Values represent the mean±s.d. of data (n=3 per group). (d) Quantification of apoptotic cell death in heart tissue. The serial sections of tissues fromcwere examined for apoptotic cell death by immunohistochemical staining using antibody that binds to cleaved (active) caspase-3. The active caspase-3-positive cells in a whole longitudinal tissue section were counted. Values represent the mean±s.d. of data (n=5 per group).Pvalues were determined by Wilcoxon rank sum test. CON, control. Full size image Figure 2: Cardiac hypertrophy in RagA/B cKO mice. ( a ) Images of wheat germ agglutinin (WGA)-stained heart tissues. Representative images from control and RagA/B cKO tissues are shown. Scale bars, 100 μm. ( b ) Cross-sectional area of cardiomyocytes. The area of cardiomyocytes from a was measured using the ImageJ software. Values represent the mean±s.d. of data ( n =15 per group). ( c ) Quantification of cell proliferation in heart tissues. Longitudinal sections of whole mount of hearts were stained with phsopho-Histone3 (p-H3) antibody to detect proliferating cardiomyocytes. The p-H3-positive cells in a whole longitudinal tissue section were counted. Values represent the mean±s.d. of data ( n =3 per group). ( d ) Quantification of apoptotic cell death in heart tissue. The serial sections of tissues from c were examined for apoptotic cell death by immunohistochemical staining using antibody that binds to cleaved (active) caspase-3. The active caspase-3-positive cells in a whole longitudinal tissue section were counted. Values represent the mean±s.d. of data ( n =5 per group). P values were determined by Wilcoxon rank sum test. CON, control. Full size image The difference of heart size between RagA/B cKO mice and control littermates was easily noticeable, and both left (LVs) and right ventricles were highly dilated in RagA/B cKO hearts ( Fig. 1b ). Consistent with the increased heart size, the heart/body weight index of RagA/B cKO mice was significantly increased compared with the control mice ( Fig. 1c ), whereas the body weight of RagA/B cKO mice was not significantly different from the control littermates. In addition, we found that the RagA/B cKO mice displayed a premature sudden death phenotype ( Fig. 1d ). Fifty percent of RagA/B cKO mice died at 7–8 months, but did not show any noticeable signs of illness or pain-like hunched position or impaired motor activity before the death. Meanwhile, the weight of lung and liver tissues was not affected in RagA/B cKO mice ( Fig. 1e,f ), thereby suggesting a relatively compensated haemodynamic state with no clear signs of overt heart failure. Because an increase of cell size and/or cell proliferation could contribute to organ size, we investigated which factors could have contributed to the heart enlargement. We compared the size of RagA/B cKO cardiomyocytes with control cardiomyocytes using heart tissue sections stained with wheat germ agglutinin ( Fig. 2a ). The cell size measurement showed that the RagA/B cKO cardiomyocytes are almost three times larger when compared with control cardiomyocytes ( Fig. 2b ). Although a cell proliferation marker, phospho-Histone3 (p-H3) staining showed a slight increase ( P =0.077, Wilcoxon rank sum test) of p-H3-positive cells in RagA/B cKO hearts despite few overall proliferating cells in a whole longitudinal section ( Fig. 2c ). Since there was a marginal increase ( P =0.075) of cleaved caspase-3-positive cells in RagA/B cKO hearts ( Fig. 2d ) and the RagA/B cKO hearts displayed massive degeneration (see below), the increased number of proliferating cells in RagA/B cKO hearts may be because of a regeneration or repair process of the cardiac muscle [26] . Therefore, we conclude that the cardiac enlargement of RagA/B cKO mice is resulted from the cellular hypertrophy of cardiomyocytes. Of note, the single conditional KO of either RagA or RagB in cardiomyocytes was not sufficient to induce cardiac enlargement ( Fig. 3a ), further supporting a functional redundancy of RagA and RagB in the heart. Thus, the heart/body weight index of the single conditional KO mice was not different from the control littermates ( Fig. 3b ), and mTORC1 signalling was not altered in the single KO mice ( Fig. 3c ). Despite the dominant RagA expression in the heart, RagB protein level was not changed upon RagA deletion ( Fig. 3c ). 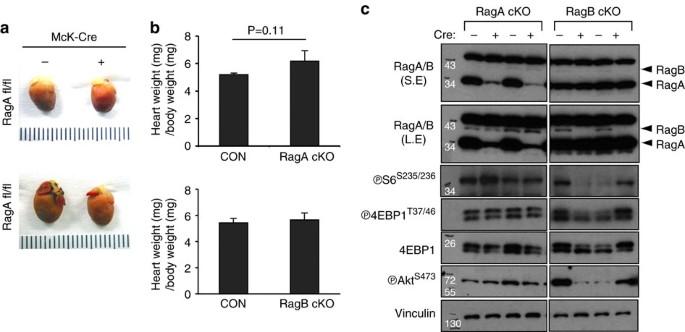Figure 3: RagA or RagB single conditional KO in heart does not cause cardiac hypertrophy. (a) Representative images of whole-mount hearts. Hearts were isolated from Mck-Cre/+;RagA flox/flox (2 months old) or Mck-Cre/+;RagB flox/flox (3 months old) mice, and the size of heart was compared with control littermates. (b) Heart/body weight index. Heart weight was divided by body weight. Values represent the mean±s.d. of data (n=3 per group).Pvalues were determined by signed rank test. (c) Immunoblot analysis using heart tissue lysates. Tissue lysates from control, RagA or RagB single cKO hearts were analysed by immunoblotting using the indicated antibodies. CON, control; S.E., short exposure; L.E., long exposure. Figure 3: RagA or RagB single conditional KO in heart does not cause cardiac hypertrophy. ( a ) Representative images of whole-mount hearts. Hearts were isolated from Mck-Cre/+;RagA flox/flox (2 months old) or Mck-Cre/+;RagB flox/flox (3 months old) mice, and the size of heart was compared with control littermates. ( b ) Heart/body weight index. Heart weight was divided by body weight. Values represent the mean±s.d. of data ( n =3 per group). P values were determined by signed rank test. ( c ) Immunoblot analysis using heart tissue lysates. Tissue lysates from control, RagA or RagB single cKO hearts were analysed by immunoblotting using the indicated antibodies. CON, control; S.E., short exposure; L.E., long exposure. Full size image RagA/B cKO causes heart dysfunction and cardiomyopathy We further examined the pathological features of the cardiac hypertrophy in RagA/B cKO mice. Histological analysis demonstrated characteristics of cardiomyopathy in RagA/B cKO hearts, including myocyte disarray and nuclear enlargement ( Fig. 4a , refer to arrows). Furthermore, vacuole formation was prevalent (arrowheads in Fig. 4a ), and fibrosis was evident by the positive trichrome staining in 1-year-old mice ( Fig. 4a , bottom panel). 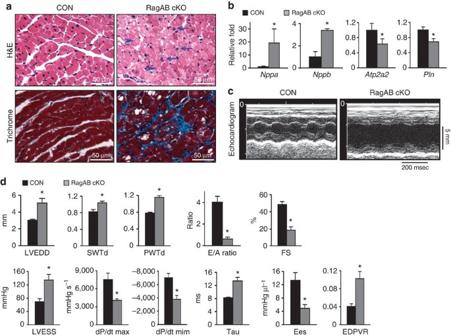Figure 4: Characterization of the cardiac hypertrophy in RagA/B cKO mice. (a) Images of haematoxylin and eosin (H&E; top, 2-month-old mice) or Masson’s trichrome (bottom, 1-year-old mice)-stained heart tissues. Arrows and arrowheads point enlarged nuclei and vacuole formation, respectively. Representative images are shown. Scale bars, 50 μm. (b) Molecular markers of cardiac remodelling in RagA/B cKO hearts. mRNA levels of indicated genes were determined by qRT–PCR. Values represent the mean±s.d. of data (n=4 per group). (c) Images of echocardiography. Representative images of tracing are shown. (d) Measurements of echocardiography and parameters of haemodynamic analyses. LVEDD, LV end-diastolic diameter; SWTd, diastolic septal wall thickness; PWTd, diastolic posterior wall thickness; E/A ratio, early to late ventricular filling velocity; FS, fractional shortening; LVESS, LV end-systolic stress; dP/dtmax and min, the rate of LV pressure rise in systole and diastole, respectively; Ees, end-systolic elastance; EDPVR, end-diastolic pressure–volume relation slope. Values represent the mean±s.e. of data (n=4 or 5 per group). *P<0.05, Wilcoxon rank sum test. CON, control. Figure 4: Characterization of the cardiac hypertrophy in RagA/B cKO mice. ( a ) Images of haematoxylin and eosin (H&E; top, 2-month-old mice) or Masson’s trichrome (bottom, 1-year-old mice)-stained heart tissues. Arrows and arrowheads point enlarged nuclei and vacuole formation, respectively. Representative images are shown. Scale bars, 50 μm. ( b ) Molecular markers of cardiac remodelling in RagA/B cKO hearts. mRNA levels of indicated genes were determined by qRT–PCR. Values represent the mean±s.d. of data ( n =4 per group). ( c ) Images of echocardiography. Representative images of tracing are shown. ( d ) Measurements of echocardiography and parameters of haemodynamic analyses. LVEDD, LV end-diastolic diameter; SWTd, diastolic septal wall thickness; PWTd, diastolic posterior wall thickness; E/A ratio, early to late ventricular filling velocity; FS, fractional shortening; LVESS, LV end-systolic stress; d P /d t max and min, the rate of LV pressure rise in systole and diastole, respectively; Ees, end-systolic elastance; EDPVR, end-diastolic pressure–volume relation slope. Values represent the mean±s.e. of data ( n =4 or 5 per group). * P <0.05, Wilcoxon rank sum test. CON, control. Full size image Functional failure of heart is associated with the up- or downregulation of particular biomarkers. Quantitative reverse transcription (qRT)–PCR analysis demonstrated a typical profile of cardiac remodelling markers in RagA/B cKO hearts ( Fig. 4b ). Both natriuretic peptide A ( Nppa ) and natriuretic peptide B ( Nppb ) mRNA levels were upregulated, indicating increased heart wall stress. In contrast, the cardiac muscle calcium pump, sarcoplasmic reticulum calcium ATPase 2 ( Atp2a2 ), and its regulator phospholamban ( Pln ), were downregulated. Consistently, echocardiography and haemodynamic analyses showed severe LV dilation and contractile dysfunction of RagA/B cKO hearts ( Fig. 4c,d ). Specifically, the LV end-diastolic diameter (LVEDD), diastolic septal/posterior wall thickness and LV end-systolic stress were significantly increased in RagA/B cKO hearts. Meanwhile, both haemodynamic and echocardiographic parameters of systolic function were altered in RagA/B cKO mice with respect to control mice. Fractional shortening (FS), d P /d T and the end-systolic elastance (Ees) were significantly reduced in the cKO mice. Diastolic function also appeared to be decreased in RagA/B cKO mice as compared with controls: E/A ratio and –dP/dT were significantly decreased, whereas Tau and the end-diastolic pressure–volume relation slope were significantly increased. Taken together, these data show that RagA/B cKO display eccentric hypertrophy with severe reduction of cardiac function. Defective autophagy flux in RagA/B KO cells To determine the molecular mechanism of the cardiac hypertrophy, we investigated whether mTORC1 pathway was dysregulated in RagA/B cKO hearts ( Fig. 5a ). Interestingly, the downstream targets of mTORC1, S6 and 4EBP1 phosphorylation levels were slightly increased in RagA/B cKO hearts, suggesting that mTORC1 activation was not severely impaired by the loss of RagA/B in vivo . Immunohistochemical staining confirmed that the cardiomyocytes of RagA/B cKO mice maintained the level of S6 phosphorylation, suggesting that mTORC1 activity was not significantly compromised ( Fig. 5b ). These observations also suggest an alternative mechanism in mTORC1 activation in the absence of RagA/B. Further analyses using another group of mice showed that the mTORC1 activation status in the heart varied among individual mice, but was not abnormally altered in the RagA/B cKO hearts ( Supplementary Fig. 3 ). Interestingly the phospho-Akt S473 level was increased in the RagA/B cKO hearts, suggesting that either the negative feedback loop of mTORC1 to mTORC2 was deregulated or the growth factor-Akt signalling axis was upregulated to compensate for the impaired cardiomyocytes in the RagA/B cKO hearts. 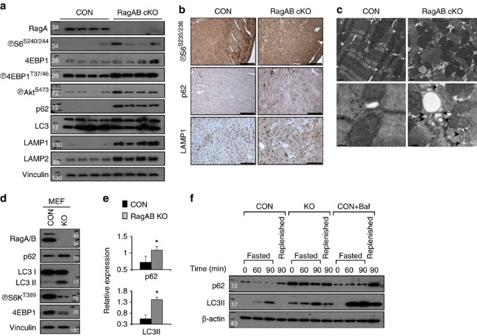Figure 5: Defective autophagy flux in RagA/B cKO hearts and MEFs (a) Immunoblot analysis using heart tissue lysates. Tissue lysates from control or RagA/B cKO hearts were analysed by immunoblotting using the indicated antibodies. (b) Immunohistochemical analysis of heart tissues. Heart tissue sections were analysed by immunohistochemistry using the indicated antibodies. Representative images are shown. Scale bars, 200 μm (S6S235/236and p62); 50 μm (LAMP1). (c) TEM of heart tissues. The ultrastructure of control and RagA/B cKO hearts was examined by TEM. Arrows and arrowheads indicate accumulation of initial autophagic vacuoles and late autophagic vacuoles/autolysosomes, respectively. Asterisks point the electron-lucent spaces. Scale bars, 1 μm (top panel); and 200 nm (bottom panel). (d) Immunoblot analysis of control and RagA/B KO MEFs. Cells were cultured in a nutrient-rich condition, and then cell lysates were analysed by immunoblotting with the indicated antibodies. (e) Quantification of immunoblot data. Levels of p62 and LC3-II were determined by densitometry. Values represent the mean±s.d. of data (n=3). *P<0.05, Wilcoxon rank sum test. (f) Immunoblot analysis of autophagy flux. Cells were cultured in a nutrient-rich medium, and then incubated in HBSS to induce autophagy. For the replenished samples, cells were re-incubated for another 90 min in a nutrient-rich medium after 90 min of starvation. A set of control cells was cultured in the presence of bafilomycin-A1(100 nM). Cell lysates were prepared at the indicated time points and analysed by immunoblotting. CON, control MEFs; KO, RagA/B KO MEFs; Baf, bafilomycin-A1. Figure 5: Defective autophagy flux in RagA/B cKO hearts and MEFs ( a ) Immunoblot analysis using heart tissue lysates. Tissue lysates from control or RagA/B cKO hearts were analysed by immunoblotting using the indicated antibodies. ( b ) Immunohistochemical analysis of heart tissues. Heart tissue sections were analysed by immunohistochemistry using the indicated antibodies. Representative images are shown. Scale bars, 200 μm (S6S 235/236 and p62); 50 μm (LAMP1). ( c ) TEM of heart tissues. The ultrastructure of control and RagA/B cKO hearts was examined by TEM. Arrows and arrowheads indicate accumulation of initial autophagic vacuoles and late autophagic vacuoles/autolysosomes, respectively. Asterisks point the electron-lucent spaces. Scale bars, 1 μm (top panel); and 200 nm (bottom panel). ( d ) Immunoblot analysis of control and RagA/B KO MEFs. Cells were cultured in a nutrient-rich condition, and then cell lysates were analysed by immunoblotting with the indicated antibodies. ( e ) Quantification of immunoblot data. Levels of p62 and LC3-II were determined by densitometry. Values represent the mean±s.d. of data ( n =3). * P <0.05, Wilcoxon rank sum test. ( f ) Immunoblot analysis of autophagy flux. Cells were cultured in a nutrient-rich medium, and then incubated in HBSS to induce autophagy. For the replenished samples, cells were re-incubated for another 90 min in a nutrient-rich medium after 90 min of starvation. A set of control cells was cultured in the presence of bafilomycin-A 1 (100 nM). Cell lysates were prepared at the indicated time points and analysed by immunoblotting. CON, control MEFs; KO, RagA/B KO MEFs; Baf, bafilomycin-A 1 . Full size image Inhibition of autophagy flux is known to cause cardiac hypertrophy in mice [27] , [28] , and the Rag GTPases localize lysosomes that have critical roles in autophagy flux. Thus, we examined whether the autophagy flux was affected in RagA/B cKO hearts. The conversion of LC3-I to LC3-II (a lipidated form of LC3) is commonly used as a marker for autophagy induction, whereas the degradation of p62 is used to measure protein degradation by autophagy flux. Interestingly, p62 protein was abnormally accumulated in RagA/B cKO hearts even though the level of LC3 lipidation was not significantly different from that of control hearts ( Fig. 5a,b ). These results suggest that autophagy initiation (autophagosome formation) may not be significantly altered while autolysosomal degradation is blocked in RagA/B cKO hearts [29] . In addition, the lysosomal marker proteins, lysosome-associated membrane protein-1 (LAMP1) and LAMP2, were abnormally accumulated in RagA/B cKO hearts ( Fig. 5a,b ). We further assessed the ultrastructure of cardiomyocytes in tissue sections using transmission electron microscopy (TEM; Fig. 5c and Supplementary Fig. 4A–F ). RagA/B cKO cardiomyocytes displayed degeneration and myofibril disarray. Consistent with the observed vacuoles in histological analysis ( Fig. 4a ), there were many electron-lucent spaces in the cytoplasm of RagA/B cKO myocytes (asterisks in Fig. 5c and Supplementary Fig. 4A–F ). Moreover, they were associated with accumulation of initial autophagic vacuoles (arrows) and late (degradative) autophagic vacuoles/autolysosomes (arrowheads in Fig. 5c and Supplementary Fig. 4A–F ) [29] . Accordingly, these data indicate that autophagosomes and autolysosomes are abnormally accumulated in RagA/B cKO hearts. Because the autophagy flux is a very dynamic process and it is difficult to manipulate the process in vivo , we used RagA and RagB double KO mouse embryonic fibroblast cells (RagA/B KO MEFs) for further investigation. First, we performed immunoblot analysis using cells that were cultured in nutrient-rich conditions ( Fig. 5d ). Both RagA and RagB proteins were absent in RagA/B KO MEFs, and phosphorylation of the mTORC1 substrates, S6K and 4EBP1, was decreased but not abolished. Interestingly, both p62 and LC3-II levels were increased about two- and threefold, respectively, in RagA/B KO MEFs compared with control cells ( Fig. 5e ). To compare the autophagy flux of RagA/B KO MEFs with that of control cells under different nutrient conditions, cells were fasted with the Hank’s balanced salt solution (HBSS) for 60 or 90 min, and then cultured in a nutrient-rich medium for 90 min ( Fig. 5f ). Again, the basal LC3-II level was higher in RagA/B KO MEFs compared with control cells under normal conditions (time 0). LC3-II levels were further increased upon fasting in both wild-type and RagA/B KO MEFs, suggesting that the LC3 lipidation and autophagy initiation were normally induced in the KO cells. Consistently, rapamycin, an mTOR inhibitor treatment further increased the LC3-II formation in the RagA/B KO MEFs under the nutrient-rich condition ( Supplementary Fig. 4G ). These data show a tight inverse correlation between mTORC1 activity and LC3-II formation. Thus, the elevated basal LC3-II formation in the KO MEFs was probably because of, at least in part, the reduced mTORC1 activity in these cells. Meanwhile, LC3-II in RagA/B KO MEFs did not disappear after the cells were replenished with a nutrient-rich medium, whereas LC3-II disappeared in control MEFs under the same treatment ( Fig. 5f ). Taken together, these data indicate that autophagy initiation can still be stimulated by nutrient deprivation in the RagA/B KO cells. However, p62 protein level was maintained at a higher level and remained even under starvation conditions in RagA/B KO MEFs despite more LC3 lipidation, suggesting that degradation of p62 was uncoupled from LC3-II accumulation (autophagy induction) in RagA/B KO MEFs. Of note, accumulation of both p62 protein and LC3-II in RagA/B KO MEFs was similar to the control MEFs treated with bafilomycin-A 1 , a v-ATPase inhibitor that blocks autophagy flux by inhibiting lysosomal acidification ( Fig. 5f ). Furthermore, we also observed that bafilomycin-A 1 treatment during autophagy flux did not further increase the accumulation of p62 and LC3-II in the RagA/B KO MEFs ( Supplementary Fig. 4H ). Taken together, these results support a model that the late stage of autophagy flux, autolysosomal degradation is likely compromised in RagA/B KO MEFs. Altered expression of lysosomal proteins in RagA/B KO MEFs Recent studies showed that TFEB is a master regulator of lysosome biogenesis and autophagy by stimulating expression of many lysosomal and autophagy related genes [15] . TFEB function is regulated by nutrients, and its nuclear localization is inhibited by mTORC1 and Rag GTPases [16] , [17] , [30] . Interestingly, the levels of the lysosomal marker LAMP1 and LAMP2 were increased in RagA/B cKO hearts ( Fig. 5a ). Accordingly, we explored the possibility that deregulation of TFEB in RagA/B KO MEFs may contribute to lysosomal dysfunction. At first, control and RagA/B KO MEFs were infected with recombinant retroviruses expressing GFP (green fluorescent protein)-tagged TFEB (TFEB-GFP), and then the localization of TFEB was investigated under either nutrient-rich conditions or starvation conditions ( Fig. 6a ). As expected, TFEB-GFP protein was exclusively localized in the cytoplasm under nutrient-rich conditions that promoted high mTORC1 activity as indicated by the positive staining for phospho-S6 S235/236 . TFEB-GFP was translocated to the nucleus in control MEFs under starvation conditions (2 h in HBB solution). In contrast, TFEB-GFP protein was localized in the nucleus in RagA/B KO MEFs regardless of nutrient conditions and even in the phospho-S6 S235/236 -positive cells (arrows, Fig. 6a ). These data show that TFEB is constitutively active in RagA/B KO cells regardless of the mTORC1 activation status. 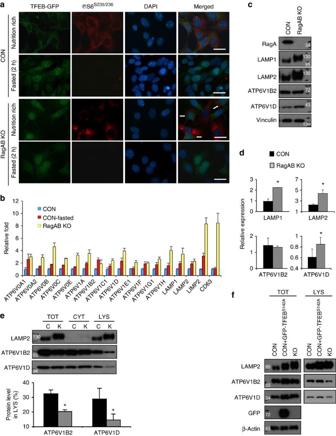Figure 6: Altered lysosomal protein expression in RagA/B KO MEFs. (a) Nuclear localization of TFEB in RagA/B KO MEFs. TFEB-GFP expressing control or RagA/B KO MEFs were cultured either in a nutrient-rich medium or in HBSS for 2 h, and then cells were fixed to examine the localization of TFEB-GFP proteins and immuno-stained with phospho-S6S235/236antibody. Representative images are shown. Scale bars, 50 μm. (b) qRT–PCR of v-ATPase subunits and lysosomal membrane proteins. Total RNAs were prepared from control, 2 h-fasted control, or RagA/B KO MEFs, and the expression levels of indicated genes were determined. (c) Immunoblot analysis of v-ATPase subunits and lysosomal membrane proteins. The levels of lysosomal membrane proteins and v-ATPase subunits were compared by immunoblotting. (d) Quantification of immunoblot analysis by densitometry. (e) The levels of v-ATPase subunits in lysosome fraction. Cell lysates were fractionated, and the amounts of v-ATPase subunits in each fraction were compared between control and RagA/B KO MEFs. The loading amount of cell lysates was normalized with ATP6V1D, and the percentage of the v-ATPase subunit level in lysosome fraction was determined by densitometric analysis. (f) Comparison of the lysosomal v-ATPase level in TFEBS142Aexpressing cells. The amounts of LAMP2, ATP6V1B2 and ATP6V1D in total or lysosomal fraction of GFP-TFEBS142Aexpressing cells were compared with control and RagA/B KO MEFs. For the lysosomal fraction, the protein loading amounts were normalized with LAMP2 levels. DAPI, 4′,6-diamidino-2-phenylindole; C, control MEFs; K, RagA/B KO MEFs; TOT, total; CYT, cytosolic fraction; LYS, lysosome fraction. All values represent the mean±s.d. of data (n=3 per group). *P<0.05, Wilcoxon rank sum test. Figure 6: Altered lysosomal protein expression in RagA/B KO MEFs. ( a ) Nuclear localization of TFEB in RagA/B KO MEFs. TFEB-GFP expressing control or RagA/B KO MEFs were cultured either in a nutrient-rich medium or in HBSS for 2 h, and then cells were fixed to examine the localization of TFEB-GFP proteins and immuno-stained with phospho-S6 S235/236 antibody. Representative images are shown. Scale bars, 50 μm. ( b ) qRT–PCR of v-ATPase subunits and lysosomal membrane proteins. Total RNAs were prepared from control, 2 h-fasted control, or RagA/B KO MEFs, and the expression levels of indicated genes were determined. ( c ) Immunoblot analysis of v-ATPase subunits and lysosomal membrane proteins. The levels of lysosomal membrane proteins and v-ATPase subunits were compared by immunoblotting. ( d ) Quantification of immunoblot analysis by densitometry. ( e ) The levels of v-ATPase subunits in lysosome fraction. Cell lysates were fractionated, and the amounts of v-ATPase subunits in each fraction were compared between control and RagA/B KO MEFs. The loading amount of cell lysates was normalized with ATP6V1D, and the percentage of the v-ATPase subunit level in lysosome fraction was determined by densitometric analysis. ( f ) Comparison of the lysosomal v-ATPase level in TFEB S142A expressing cells. The amounts of LAMP2, ATP6V1B2 and ATP6V1D in total or lysosomal fraction of GFP-TFEB S142A expressing cells were compared with control and RagA/B KO MEFs. For the lysosomal fraction, the protein loading amounts were normalized with LAMP2 levels. DAPI, 4′,6-diamidino-2-phenylindole; C, control MEFs; K, RagA/B KO MEFs; TOT, total; CYT, cytosolic fraction; LYS, lysosome fraction. All values represent the mean±s.d. of data ( n =3 per group). * P <0.05, Wilcoxon rank sum test. Full size image To determine the transcriptional activity of TFEB in control and RagA/B KO MEFs, we measured the expression of TFEB target genes by qRT–PCR ( Fig. 6b ). We assessed a subset of known TFEB direct target genes, including some v-ATPase subunits and lysosomal membrane proteins, because they are essential for lysosomal acidification and function [31] , [32] , [33] . As expected, most of the TFEB target genes were upregulated by starvation in control MEFs ( Fig. 6b ). We also found that all TFEB target genes tested were significantly upregulated in RagA/B KO MEFs compared with control MEFs under nutrient-rich conditions, further supporting the constitutive activation of TFEB in RagA/B KO MEFs. We next compared the protein levels of TFEB target genes using immunoblotting analysis ( Fig. 6c ). Consistent with the qRT-PCR data, the protein levels of LAMP1 and LAMP2 were about twofold more abundant in the RagA/B KO MEFs than the control MEFs. However, the v-ATPase subunit ATP6V1B2 protein level was not changed, whereas another v-ATPase subunit ATP6V1D protein level was marginally (~50%) increased in RagA/B KO MEFs ( Fig. 6d ). Thus, these data indicate that the molecular ratio between the lysosomal membrane proteins and v-ATPase subunits is altered in RagA/B KO MEFs. v-ATPase can localize on intracellular vesicular membranes and the plasma membrane. Lysosomal localization of the v-ATPase is required to acidify lysosomes. Therefore, we investigated whether the altered expression of lysosomal proteins affects the level of v-ATPase on lysosomes in RagA/B KO MEFs. We fractionated cells into cytoplasm and lysosome fractions, and examined the v-ATPase distribution ( Fig. 6e , the total protein loading amounts were normalized with ATP6V1D levels). We found that the levels of both ATP6V1B2 and ATP6V1D protein in the lysosome fraction were significantly lower in RagA/B KO MEFs compared with control cells, and the relative ratio of v-ATPase subunits to the lysosomal membrane protein LAMP2 was decreased in RagA/B KO cells. Quantification analysis revealed that only ~15–20% of total ATP6V1B2 and ATP6V1D was co-isolated in the lysosome fraction of RagA/B KO MEFs, whereas ~30–33% of those proteins resided in the lysosome fraction of control MEFs. These data are intriguing because it has been shown that the activation of TFEB facilitates autophagy flux and lysosomal function [18] , [19] , [20] . Therefore, we further investigated whether constitutive activation of TFEB contributed to the decreased v-ATPase expression in the lysosome fraction. Overexpression of a constitutively active mutant TFEB (TFEB S142A ) [18] in control MEFs upregulated both LAMP2 and ATP6V1D protein levels similar to those in the RagA/B KO cells, supporting the notion that RagA/B regulate lysosomal protein expression via TFEB. However, the lysosomal localization of ATP6V1B2 and ATP6V1D in the TFEB S142A expressing cells was still higher than the RagA/B KO MEFs ( Fig. 6f , the lysosome fractions were normalized with LAMP2 levels), indicating that RagA/B influence v-ATPase localization independent of TFEB. Taken together, our data suggest that the Rag GTPases modulate lysosomal function, at least in part, by affecting lysosomal protein expression and localization. In order to determine whether the decreased lysosomal v-ATPase expression in RagA/B KO MEFs can be restored by RagA, the RagA/B KO MEFs were infected with RagA-encoding recombinant retroviruses. Re-introduction of RagA in the RagA/B KO MEFs not only restored both ATP6V1B2 and ATP6V1D levels in the lysosome fraction, but also rescued the defects of autophagy flux ( Fig. 7a–c , the fractionated samples were normalized with LAMP2 level). Furthermore, to investigate whether the diminished mTORC1 activity affected the lysosomal v-ATPase localization in RagA/B KO MEFs, we also generated RagA/B KO MEF cell lines expressing either Rheb WT or constitutively active Rheb (Rheb S16H ). Despite substantial restoration of mTORC1 activity by Rheb WT or Rheb S16H as indicated by increased S6K1 phosphorylation ( Fig. 7d ), the total LAMP2 protein level and lysosomal ATP6V1B2 localization were not restored to normal ( Fig. 7e ). Moreover, autophagy flux was not recovered in Rheb S16H expressing RagA/B KO MEFs ( Fig. 7f ). We also examined whether mTORC1 inactivation by either nutrient deprivation or dominant-negative RagA (RagA TN ) expression in control MEFs affects lysosomal v-ATPase localization. The expression of RagA TN did not completely inhibit mTORC1 probably owing to insufficient expression level and had no substantial effect on the lysosomal localization of v-ATPase. Intriguingly, the nutrient deprivation also did not affect the lysosomal v-ATPase localization despite of complete mTORC1 inactivation ( Fig. 7g ). Collectively, these data indicate that the Rag GTPases modulate the lysosomal v-ATPase localization independent of mTORC1 activity. 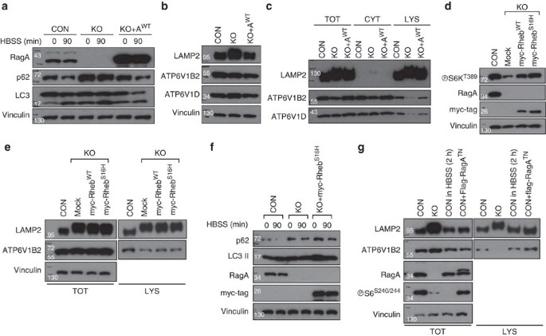Figure 7: Restored autophagy flux and lysosomal v-ATPase localization in RagA/B KO MEFs by RagAWTexpression, but not by RhebWTor RhebS16Hexpression. (a) Restoration of autophagy flux in RagA/B KO MEFs by reintroducing RagAWT. RagA/B KO MEFs were infected with wild-type RagA (RagAWT) expressing retroviruses, and then autophagy flux was examined by immunoblotting. (b) Immunoblot analysis of TFEB target gene expression. The expression levels of LAMP2, ATP6V1B2 and ATP6V1D were restored by RagAWTexpression in the RagA/B KO MEFs. (c) Immunoblot analysis of lysosomal v-ATPase subunits. Cells were fractionated, and the levels of v-ATPase subunits in total, cytoplasm and lysosomal fraction were examined by immunoblotting. The protein loading amounts were normalized with LAMP2 protein levels. (d) RhebWTor RhebS16Hexpression substantially restores mTORC1 activity in RagA/B KO MEFs. Stable cell lines were generated by infecting RagA/B KO MEFs with RhebWTor RhebS16Hencoding retroviruses, and then cell lysates were analysed by immunoblotting. (e) RhebWTor RhebS16Hdoes not restore lysosomal v-ATPase localization in RagA/B KO MEFs. Cells were fractionated, and the lysates were analysed by immunoblotting. (f) Immunoblot analysis of autophagy flux. Cells were cultured in a nutrient-rich medium followed by starvation in HBSS for 90 min, and autophagy flux markers were examined by immunoblotting. (g) Nutrient deprivation or RagATNexpression in control MEFs does not alter lysosomal v-ATPase localization. Starved control MEFs (in HBSS for 2 h) or RagATNexpressing control MEFs were fractionated and analysed by immunoblotting. CON, control MEFs; KO, RagA/B KO MEFs; AWT, RagA wild-type; TOT, total; CYT, cytoplasm; LYS, lysosome fraction. Figure 7: Restored autophagy flux and lysosomal v-ATPase localization in RagA/B KO MEFs by RagA WT expression, but not by Rheb WT or Rheb S16H expression. ( a ) Restoration of autophagy flux in RagA/B KO MEFs by reintroducing RagA WT . RagA/B KO MEFs were infected with wild-type RagA (RagA WT ) expressing retroviruses, and then autophagy flux was examined by immunoblotting. ( b ) Immunoblot analysis of TFEB target gene expression. The expression levels of LAMP2, ATP6V1B2 and ATP6V1D were restored by RagA WT expression in the RagA/B KO MEFs. ( c ) Immunoblot analysis of lysosomal v-ATPase subunits. Cells were fractionated, and the levels of v-ATPase subunits in total, cytoplasm and lysosomal fraction were examined by immunoblotting. The protein loading amounts were normalized with LAMP2 protein levels. ( d ) Rheb WT or Rheb S16H expression substantially restores mTORC1 activity in RagA/B KO MEFs. Stable cell lines were generated by infecting RagA/B KO MEFs with Rheb WT or Rheb S16H encoding retroviruses, and then cell lysates were analysed by immunoblotting. ( e ) Rheb WT or Rheb S16H does not restore lysosomal v-ATPase localization in RagA/B KO MEFs. Cells were fractionated, and the lysates were analysed by immunoblotting. ( f ) Immunoblot analysis of autophagy flux. Cells were cultured in a nutrient-rich medium followed by starvation in HBSS for 90 min, and autophagy flux markers were examined by immunoblotting. ( g ) Nutrient deprivation or RagA TN expression in control MEFs does not alter lysosomal v-ATPase localization. Starved control MEFs (in HBSS for 2 h) or RagA TN expressing control MEFs were fractionated and analysed by immunoblotting. CON, control MEFs; KO, RagA/B KO MEFs; A WT , RagA wild-type; TOT, total; CYT, cytoplasm; LYS, lysosome fraction. Full size image Given the fact that TFEB regulates p62 expression [18] and its constitutive activation in RagA/B KO MEFs, we examined whether the amount of p62 mRNA in the KO MEFs or TFEB S142A expressing control MEFs were upregulated. qRT-PCR analyses showed that p62 mRNA levels were about 1.7- and 3.5-fold increased in the RagAB KO MEFs and TFEB S142A expressing cells, respectively ( Fig. 8a ). However, nutrient starvation could substantially decrease p62 protein in both the control and the TFEB S142A expressing MEFs, but not in the RagA/B KO MEFs ( Fig. 8b ). As expected, p62 levels were higher in the TFEB S142A MEFs likely due to enhanced transcription. These data indicate that both the defective autolysosomal degradation and transcriptional upregulation contribute to the increased level of p62 in the RagA/B KO MEFs. 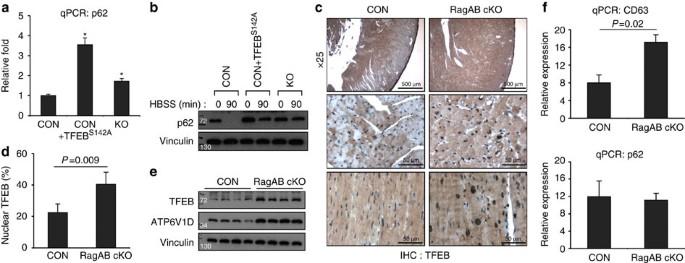Figure 8: Increased TFEB activity in RagA/B KO MEFs and RagA/B cKO hearts. (a) p62 mRNA levels were upregulated in RagA/B KO MEFs and TFEBS142Aexpressing control MEFs. Total RNAs were prepared from cells and p62 mRNA levels were quantified using qPCR. Values represent mean±s.d. of data (n=4 per group). *Pvalue=0.021. (b) Immunoblot analysis of p62 degradation by starvation. p62 levels were substantially decreased in control and TFEBS142Aexpressing control MEFs by starvation (in HBSS for 90 min), but not in RagA/B KO MEFs. (c) Immunohistochemical analyses of heart tissues using TFEB antibody. Top panel, low magnification view shows uneven distribution of TFEB expression in the control hearts (scale bars, 500 μm). Middle panel, high magnification view of LV wall areas (scale bars, 50 μm). Bottom panel, inter-ventricular septum areas (scale bars, 50 μm). (d) Quantification of TFEB-positive nuclei. The number of TFEB-positive nuclei were divided by total number of nuclei per microscopic field. Values represent mean±s.d. of data (n=5 per group). (e) Immunoblot analysis of heart tissue lysates. TFEB and its target ATP6V1D levels were upregulated in RagA/B cKO hearts compared with controls. (f) qRT–PCR analyses of TFEB target genes from heart tissues. Total RNAs were prepared from heart tissues, and mRNA levels of TFEB target genes,CD63andp62, were quantified by qPCR. Values represent mean±s.d. of data (n=4 per group).Pvalues were determined by Wilcoxon rank sum test. CON, control. Figure 8: Increased TFEB activity in RagA/B KO MEFs and RagA/B cKO hearts. ( a ) p62 mRNA levels were upregulated in RagA/B KO MEFs and TFEB S142A expressing control MEFs. Total RNAs were prepared from cells and p62 mRNA levels were quantified using qPCR. Values represent mean±s.d. of data ( n =4 per group). * P value=0.021. ( b ) Immunoblot analysis of p62 degradation by starvation. p62 levels were substantially decreased in control and TFEB S142A expressing control MEFs by starvation (in HBSS for 90 min), but not in RagA/B KO MEFs. ( c ) Immunohistochemical analyses of heart tissues using TFEB antibody. Top panel, low magnification view shows uneven distribution of TFEB expression in the control hearts (scale bars, 500 μm). Middle panel, high magnification view of LV wall areas (scale bars, 50 μm). Bottom panel, inter-ventricular septum areas (scale bars, 50 μm). ( d ) Quantification of TFEB-positive nuclei. The number of TFEB-positive nuclei were divided by total number of nuclei per microscopic field. Values represent mean±s.d. of data ( n =5 per group). ( e ) Immunoblot analysis of heart tissue lysates. TFEB and its target ATP6V1D levels were upregulated in RagA/B cKO hearts compared with controls. ( f ) qRT–PCR analyses of TFEB target genes from heart tissues. Total RNAs were prepared from heart tissues, and mRNA levels of TFEB target genes, CD63 and p62 , were quantified by qPCR. Values represent mean±s.d. of data ( n =4 per group). P values were determined by Wilcoxon rank sum test. CON, control. Full size image To examine the role of the RagA/B in TFEB regulation in vivo , we investigated nuclear TFEB localization in the RagA/B cKO heart tissue using immunohistochemistry ( Fig. 8c ). TFEB expression was not distributed evenly in control hearts, specifically lower in the ventricular wall area, whereas consistent TFEB expression was observed in RagA/B cKO hearts (top panel, Fig. 8c ). Quantitative analysis showed that the percentage of TFEB-positive nuclei per field was increased about twofold in the RagA/B cKO hearts compared with control hearts ( Fig. 8d ). Consistent with this observation, immunoblotting analyses showed that TFEB protein level and its transcriptional target ATP6V1D were increased in the RagA/B cKO hearts ( Fig. 8e ), confirming that TFEB activity was upregulated in the cKO hearts. Of note, it has been also suggested that TFEB positively regulates its own expression [34] . However, unlike RagA/B KO MEFs, p62 mRNA level was not significantly increased in the RagA/B cKO hearts even though another TFEB target gene, CD63 , was significantly upregulated ( Fig. 8f ). A possible explanation is that the elevated p62 protein in the RagA/B cKO hearts ( Fig. 5a ) might indirectly suppress its own expression. Alternatively, the high basal TFEB activity in the control hearts (nuclear TFEB signals were observed in ~20% cells, Fig. 8d ) may mask the p62 induction by the RagA/B KO-induced further activation of TFEB. Nonetheless, our data suggest that in the RagA/B cKO hearts, impaired autolysosomal degradation contributes to p62 accumulation. Lysosomal acidification is compromised in RagA/B KO MEFs The accumulation of p62 and autophagosomes in the RagA/B KO hearts and MEFs suggests a possible defect in lysosomal degradation. Acidification is critical for lysosome function and hydrolytic degradation. Therefore, we assessed the lysosomal pH in live cells to determine whether the decreased lysosomal v-ATPase level affected the pH of lysosome. The lysosomal pH of RagA/B KO MEFs was significantly higher than that of control MEFs ( Fig. 9a ), supporting the notion that the Rag GTPases have a role in lysosomal function. Some lysosomal hydrolytic enzymes are matured by a proteolytic process in a pH-dependent manner, such as cathepsin D maturation [35] . Thus, we investigated whether the maturation of cathepsin D was defective in RagA/B KO MEFs. Immunoblot analysis using the lysosome fractions (normalized with LAMP1 protein level) showed that the matured cathepsin D was significantly impaired in RagA/B KO MEFs (arrow head, Fig. 9b ), indicating defective acidification of lysosome and dysfunction. Moreover, we consistently observed that both LAMP1 and LAMP2 proteins present higher molecular weights in RagA/B KO MEFs compared with control MEFs. Multiple post-translational modifications occur in the lysosomes, and the sialylation of LAMP1 and LAMP2 are modified by lysosomal N-acetyl-α-neuraminidase (sialidase) [36] , [37] . Thus, treatment of sialidase A increased the mobility of LAMP2 in the RagA/B KO MEFs, although not to the migration of the LAMP2 in the control MEFs ( Fig. 9c ), indicating that LAMP2 proteins were over sialylated in RagA/B KO MEFs. Consistent with unchanged lysosomal v-ATPase level in TFEB S142A expressing control MEFs ( Fig. 6f ), we also observed that the maturation of cathepsin D was not impaired in those cells ( Fig. 9d ). 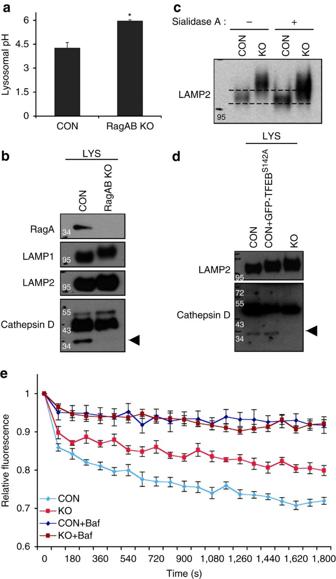Figure 9: Lysosomal acidification is compromised in RagA/B KO MEFs. (a) Lysosomal pH measurement in live cells. Cells were fed with OG541-conjugated dextran for overnight followed by serum starvation for 1 h, and then trypsinized for spectrofluorimetric measurement. Values represent the mean±s.d. of data (n=3 per group). *P<0.05, Wilcoxon rank sum test. (b) Immunoblot analysis of cathepsin D maturation in lysosome fraction. Lysosome fractions from control and RagA/B KO MEFs were analysed by immunoblotting using the indicated antibodies. The amount of protein loading was normalized with LAMP1 protein level. Arrowhead indicates the matured form of cathepsin D. (c) Sialidase A treatment increases mobility of LAMP2 on SDS–PAGE. Cell lysates were incubated with sialidase A for 3 h followed by SDS–PAGE and immunoblotting. (d) Cathepsin D maturation in GFP-TFEBS142Aexpressing cells. The amounts of matured cathepsin D in lysosomal fraction of GFP-TFEBS142Aexpressing cells were compared with control and RagA/B KO MEFs using immunoblotting. The amount of protein loading was normalized with LAMP2 protein level. Arrowhead indicates the matured form of cathepsin D. (e) A compromised lysosomal acidification capacity in RagA/B KO MEFs. Cells were fed with a pH-sensitive fluorescent dye (OG541)-conjugated dextran for overnight, and then starved in a serum-free medium for 2 h. v-ATPase-mediated acidification of LEF was measured in the absence or in the presence of bafilomycin-A1(100 nM)in vitro. The amount of lysosome fraction was normalized with LAMP2 protein level. Each point represents the mean±s.e. of three 30-s intervals from three independent measurements. CON, control MEFs; KO, RagA/B KO MEFs; Baf, bafilomycin-A1. Figure 9: Lysosomal acidification is compromised in RagA/B KO MEFs. ( a ) Lysosomal pH measurement in live cells. Cells were fed with OG541-conjugated dextran for overnight followed by serum starvation for 1 h, and then trypsinized for spectrofluorimetric measurement. Values represent the mean±s.d. of data ( n =3 per group). * P <0.05, Wilcoxon rank sum test. ( b ) Immunoblot analysis of cathepsin D maturation in lysosome fraction. Lysosome fractions from control and RagA/B KO MEFs were analysed by immunoblotting using the indicated antibodies. The amount of protein loading was normalized with LAMP1 protein level. Arrowhead indicates the matured form of cathepsin D. ( c ) Sialidase A treatment increases mobility of LAMP2 on SDS–PAGE. Cell lysates were incubated with sialidase A for 3 h followed by SDS–PAGE and immunoblotting. ( d ) Cathepsin D maturation in GFP-TFEB S142A expressing cells. The amounts of matured cathepsin D in lysosomal fraction of GFP-TFEB S142A expressing cells were compared with control and RagA/B KO MEFs using immunoblotting. The amount of protein loading was normalized with LAMP2 protein level. Arrowhead indicates the matured form of cathepsin D. ( e ) A compromised lysosomal acidification capacity in RagA/B KO MEFs. Cells were fed with a pH-sensitive fluorescent dye (OG541)-conjugated dextran for overnight, and then starved in a serum-free medium for 2 h. v-ATPase-mediated acidification of LEF was measured in the absence or in the presence of bafilomycin-A 1 (100 nM) in vitro . The amount of lysosome fraction was normalized with LAMP2 protein level. Each point represents the mean±s.e. of three 30-s intervals from three independent measurements. CON, control MEFs; KO, RagA/B KO MEFs; Baf, bafilomycin-A 1 . Full size image To determine the molecular mechanism for defects in lysosomal acidification of the RagA/B KO cells, we measured v-ATPase activity in the lysosome fraction that was loaded with pH-sensitive fluorescent dye-conjugated dextran ( Fig. 9e ). Bafilomycin-A 1 , a specific v-ATPase inhibitor, was used to confirm the specificity of the v-ATPase assay. Consistent with the altered v-ATPase protein levels, the acidification rate of lysosome from RagA/B KO MEFs was significantly reduced compared with that from control MEFs ( Fig. 9e ). These results suggest that the reduced v-ATPase activity in the lysosomes of RagA/B KO cells is responsible for the defective lysosomal acidification and dysfunction. We next accessed whether Rag GTPases might directly regulate v-ATPase activity. Addition of immuno-purified wild-type or mutant RagA proteins (and co-immunoprecipitated RagC proteins) was not able to restore the lysosomal acidification in vitro ( Supplementary Fig. 5A–D ). Altogether, our data indicate that lysosomal acidification is compromised in RagA/B KO MEFs due to the reduced lysosomal v-ATPase, and thus resulting in lysosomal dysfunction. RagA/B cKO hearts resemble LSDs Mutations in multiple genes coding for lysosomal proteins cause LSDs in humans. Cardiac hypertrophy found in both Pompe disease (acid alpha-glucosidase defect) and Danon disease (LAMP2 defect) is associated with abnormal glycogen accumulation in cardiomyocytes due to the lysosomal dysfunction [38] , [39] . In fact, we noticed that glycogen was abnormally accumulated in RagA/B cKO hearts revealed by TEM (electro-dense granules (small double arrows) in Supplementary Fig. 4A–F ), suggesting that the cardiac hypertrophy of RagA/B cKO hearts resembles LSD. We first confirmed the abnormal glycogen accumulation in RagA/B cKO heart sections by Periodic acid-Schiff staining ( Fig. 10a ). Using a biochemical assay, we found that the amount of glycogen in the RagA/B cKO heart tissues was about three times more than the controls ( Fig. 10b ). 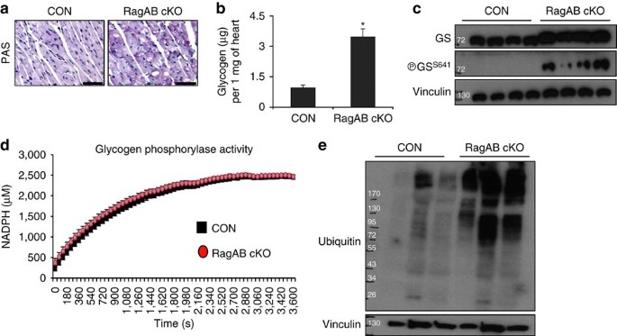Figure 10: Cardiac hypertrophy in RagA/B cKO mice exhibits the features of LSDs. (a) Periodic acid-Schiff staining of heart tissues. Representative images are shown. Scale bars, 50 μm. (b) Biochemical measurement of glycogen level in heart tissues. Glycogen levels were determined using an enzyme-based colorimetric assay kit. Values represent the mean±s.d. of data (n=4 per group). *P<0.03, Wilcoxon rank sum test. (c) Immunoblot analysis of glycogen synthase-1 in heart. Tissue lysates were prepared from control and RagA/B cKO hearts, and levels of glycogen synthase and phospho-glycogen synthase were investigated by immunoblotting. (d) Glycogen phosphorylase activity assay. Using an enzyme-based assay, activity of glycogen phosphorylase in heart tissue was determined by measuring NADPH production in the reaction. Each point represents the mean±s.d. of data (n=4 per group). (e) Accumulation of ubiquitinated proteins in RagA/B cKO hearts. Levels of ubiquitinated proteins in heart tissues were examined by immunoblotting. CON, control. Figure 10: Cardiac hypertrophy in RagA/B cKO mice exhibits the features of LSDs. ( a ) Periodic acid-Schiff staining of heart tissues. Representative images are shown. Scale bars, 50 μm. ( b ) Biochemical measurement of glycogen level in heart tissues. Glycogen levels were determined using an enzyme-based colorimetric assay kit. Values represent the mean±s.d. of data ( n =4 per group). * P <0.03, Wilcoxon rank sum test. ( c ) Immunoblot analysis of glycogen synthase-1 in heart. Tissue lysates were prepared from control and RagA/B cKO hearts, and levels of glycogen synthase and phospho-glycogen synthase were investigated by immunoblotting. ( d ) Glycogen phosphorylase activity assay. Using an enzyme-based assay, activity of glycogen phosphorylase in heart tissue was determined by measuring NADPH production in the reaction. Each point represents the mean±s.d. of data ( n =4 per group). ( e ) Accumulation of ubiquitinated proteins in RagA/B cKO hearts. Levels of ubiquitinated proteins in heart tissues were examined by immunoblotting. CON, control. Full size image Glycogen metabolism can be controlled by the classic glycogen synthase and phosphorylase. Immunoblot analysis using the heart tissue lysates showed that the glycogen synthase level was not different between control and RagA/B cKO hearts ( Fig. 10c ). Glycogen synthase activity is inhibited by phosphorylation of S641 (ref. 40 ). We found that phosphorylation of S641 in glycogen synthase was higher in RagA/B cKO hearts than the control mice, indicating that the glycogen synthase activity was repressed in the cKO heart. This is probably because of a compensatory effect of cells to counter balance the elevated glycogen level in the RagA/B cKO heart. Therefore, the abnormal glycogen accumulation could not be due to hyperactivation of glycogen synthase in the RagA/B cKO hearts. We next examined the glycogen phosphorylase, the major enzyme responsible for glycogen hydrolysis. Glycogen phosphorylase activity assays using tissue lysates demonstrated that the enzyme activity was indistinguishable between the control and the RagA/B cKO hearts ( Fig. 10d ). Altogether, these results show that the abnormal glycogen accumulation in the RagA/B cKO heart is not due to glycogen synthase or phosphorylase, but lysosomal dysfunction may be the major contributor for the glycogen accumulation. One of the hallmarks of autophagy flux defect is the accumulation of ubiquitinated proteins. Accumulation of ubiquitinated proteins is also observed in LSDs, including a mouse model of Pompe disease [14] , [41] . Consistent with the defects in autophagy flux and lysosomal function in RagA/B cKO hearts, ubiquitinated proteins were massively accumulated in RagA/B cKO heart tissues compared with control hearts ( Fig. 10e ). Collectively, these data show that the histopathological phenotype of RagA/B cKO hearts resembles the LSDs in humans. Rag GTPases are key transducers relaying amino-acid signals to cellular regulation [42] . In response to amino-acid stimulation, the Rag GTPases are activated by the Ragulator-mediated guanine nucleotide exchange and recruit mTORC1 to lysosomes via a direct binding to Raptor, a subunit of mTORC1. Rheb GTPase downstream of growth factor signalling subsequently activates the lysosomal associated mTORC1. mTORC1 has been the only well-defined physiological target of Rag GTPases in modulating cell metabolism and growth so far. In this study, we show that loss of both RagA and RagB in cardiomyocytes causes hypertrophic cardiomyopathy that resembles LSDs in humans. Notably, phosphorylation of mTORC1 downstream molecules was not significantly reduced in the RagA/B KO heart, indicating alternative mechanism or compensation for mTORC1 activation in the RagA/B KO cells. Of interest, a recent study also showed that mTORC1 can be activated regardless of nutrient levels in the absence of RagA by unknown mechanism [43] . Although further studies are necessary to elucidate the molecular mechanism of Rag GTPases-independent mTORC1 activation, our study suggests an mTORC1-independent function of Rag GTPases in regulating lysosome and autophagy flux. We propose that the defect in lysosome function and autophagy flux is responsible for the pathological phenotypes observed in the RagA/B cKO hearts. Constitutive activation of TFEB by the loss of Rag GTPases leads to excessive expression of lysosomal proteins with altered stoichiometry and decreased lysosomal localization. As a result, reduced lysosomal v-ATPase activity leads to the elevated lysosome pH and lysosomal dysfunction. Our study defines a new role of Rag GTPases in regulating lysosomal function in vivo . As an integrator of nutrient levels in the cell, mTORC1 negatively regulates autophagy initiation [44] . Because Rag GTPases mediate mTORC1 activation by nutrients, one may expect an increased autophagy flux by impaired mTORC1 activity owing to the loss of Rag GTPases. In fact, our data show that the basal level of LC3 lipidation is increased significantly in RagA/B KO MEFs even under nutrient-rich condition ( Fig. 5d,f ), suggesting that autophagy initiation is increased in the RagA/B KO cells. However, p62, which is degraded in autolysosomes at the end of autophagy flux [45] , [46] , is accumulated in the KO cells. Therefore, the simultaneous accumulation of p62 and LC3-II demonstrates a defective autophagy flux in RagA/B KO MEFs. This is consistent with the defective lysosomal function in the KO cells. Intriguingly, it has also been shown that mTORC1 regulates the reformation of lysosomes subsequent to autolysosomal degradation [47] . Currently, it is not clear whether the compromised mTORC1 activation by loss of Rag GTPases affects the reformation of lysosomes. LSDs are associated with defective autophagy flux in most cases [48] . In this study, we found that the hypertrophy of RagA/B cKO hearts displays characteristic features of LSDs: the accumulation of autophagosomes/autolysosomes, p62 protein, glycogen and ubiquitinated proteins. Therefore, our in vitro and in vivo data strongly demonstrate that loss of Rag GTPases leads to lysosomal dysfunction. The final clearance of intracellular components by autophagy requires fusion with and degradation by lysosomes. Lysosomal dysfunction is likely the cause for the defects in autophagy flux and cardiomyopathy in the RagA/B cKO heart. Our data support a critical role of autophagy in maintaining healthy cardiac function. Heart is one of the major organs affected in many LSDs, and infantile or childhood onset of Pompe disease is usually lethal due to heart failure [14] , [39] . RagA/B cKO mice also died prematurely ( Fig. 1d ). Interestingly, the mice did not show any noticeable signs of illness before death, suggesting that death may be caused predominantly by a fatal arrhythmia or, in some cases, by an acute heart failure development that immediately precedes the death. Interestingly, the lung weight was not changed in RagA/B cKO mice, suggesting that the haemodynamic state of these animals is relatively compensated despite the severe reduction of systolic function. This may be because of the activation of several known compensatory adaptations that limit the reduction of cardiac output and the increase of pulmonary vascular pressure and lung congestion in RagA/B cKO mice. RagA/B cKO mice develop extensive ventricular dilation that can partly compensate for the reduction of FS and limit the stroke volume drop. The Frank–Starling mechanism is probably still preserved in the heart of RagA/B cKO mice and it can temporarily increase the stroke volume in these animals. Chronic ventricular dilation is also known to be associated with increased ventricular compliance that would allow the ventricle of RagA/B cKO mice to have a greater end-diastolic volume without an extensive parallel increase of end-diastolic pressure. In addition, the observed increase of myocardial wall thickness and overall ventricular mass can temporarily increase ventricular contractility in RagA/B cKO mice. Finally, neurohormonal activation could also be another mechanism that would contribute to compensating the haemodynamic state of RagA/B cKO mice [49] . Recent studies have shown potential roles of Rag GTPases in lysosome function. Rag GTPases interact with v-ATPases via Ragulator [8] , [11] . Moreover, Rag GTPases directly interact with TFEB to modulate the mTORC1-mediated TFEB cytoplasmic localization [16] , [17] . TFEB is constitutively activated in the RagA/B KO cells, and as a consequence, TFEB target gene expression is significantly elevated ( Fig. 6a,b ). Despite the increased v-ATPase expression, the levels of the v-ATPase protein associated with lysosomes are actually decreased in RagA/B KO MEFs compared with control MEFs ( Fig. 6e ). As a result, lysosomal v-ATPase activity is reduced and lysosomal pH is higher ( Fig. 9 ). Consistent with this notion, maturation of lysosomal proteins, such as cathepsin D and LAMP1 and LAMP2, is impaired in the RagA/B KO cells. Intriguingly, overexpression of constitutively active mutant TFEB is not sufficient to recapitulate the RagA/B KO phenotypes ( Figs 6f and 9d ). Therefore, RagA/B modulate lysosome function in part by affecting the lysosomal localization of v-ATPase and in part by suppressing TFEB activity. VPS15 is an essential component of the VPS34 complex that is critical for autophagy induction as well as vesicular trafficking. Of note, loss of Vps15 in skeletal muscles exhibits pathological phenotypes similar to RagA/B cKO mice [50] . The Vps15 KO skeletal muscles develop autophagic vacuolar myopathy associated with accumulation of p62, autophagosomes and glycogen. Intriguingly, it has been also shown that Gtr1 and Gtr2, the yeast orthologues of Rag GTPases, regulate vesicular trafficking [4] . Therefore, Rag GTPases may regulate protein and vesicular trafficking, such as v-ATPase localization to lysosomes, by a mechanism independent of mTORC1. Future studies are necessary to gain the molecular insight of mTORC1-independent function of Rag GTPases. Generation of RagA/B conditional KO mice RagA targeting vector was constructed by inserting PCR amplified RagA gDNA fragments, including the promoter, exon and 3′ untranslated region (UTR) sequences in between two loxP sites of pflox-FRT-neo vector (Dr Ju Chen, University of California-San Diego), and the targeting vector was injected into mouse embryonic stem (ES) cells (129 SvJ) to generate RagA conditional allele ( RagA fl/+ ) by homologous recombination. G418-resistant ES cell clones were screened by Southern blotting and gDNA PCR. A targeted ES clone was injected into C57BL/6 blastocysts to generate chimeric mice. Germline transmission of RagA floxed allele of chimeric mice was confirmed by gDNA PCR genotyping, and then the chimeric mice were mated with FLPeR mice (Gt(ROSA)26Sor tm1(FLP1)Dym /J; The Jackson Laboratory) to remove neomycin-resistant gene from the targeted allele. RagB conditional allele was also generated as described above, but only the exon 3 (encodes a GDP/GTP binding site) was flanked by two loxP sites. RagA fl/+ ;RagB fl/+ mice were generated by breeding between RagA and RagB heterozygotes, and then the double heterozygote mice were intercrossed to generate the RagA fl/fl ;RagB fl/fl mice. To delete the floxed alleles in the skeletal and cardiac muscles, the single or double conditional KO mice were mated with transgenic mice expressing Cre recombinases under the control of muscle creatine kinase promoter (B6.FVB(129S4)-Tg(Ckmm-cre)5Khn/J; The Jackson Laboratory), and the offspring were backcrossed with the conditional KO mice. Therefore, the genetic background of mice is 129 SvJ and C56BL/6 mixed background, and littermates from mating of Mck-Cre /+ ; RagA fl/fl ;RagB fl/fl and RagA fl/fl ;RagB fl/fl were compared in all experiments. All animal procedures were approved by the University of California-San Diego and Rutgers New Jersey Medical School Institutional Animal Care and Use Committee and carried out in accordance with the guidelines. Generation of RagA/B KO MEFs and cell culture RagA fl/fl ;RagB fl/fl embryos were dissected out at E13.5 and trypsinized for 1 h at 37 °C. Primary MEFs were then immortalized with SV40 T antigen using a retroviral vector. The immortalized MEFs were infected with adenoviruses encoding GFP and Cre-GFP (1K MOI, Cell Biolabs, USA) to generate control and RagA/B KO MEFs, respectively. Cells were cultured in high-glucose Dulbeco's modified eagle medium (DMEM) (Invitrogen, USA) supplemented with 10% fetal bovine serum (Hyclone, USA) and antibiotics (penicillin/streptomycin). Cell fractionation Overnight cultured cells (1 × 10 6 cells on a 10-cm dish) were trypsinized and resupended in 750 μl of cold fractionation buffer (50 mM KCl, 90 mM potassium gluconate, 1 mM EGTA, 50 mM sucrose, 5 mM glucose, protease inhibitor cocktail tablet and 20 mM HEPES, pH 7.4). The cells were then lysed by sonication, and nuclear fraction was removed by centrifugation at 1,000 g for 10 min at 4 °C. The supernatant was further centrifuged at 20,000 g for 30 min at 4 °C. The precipitated lysosome-enriched fraction (LEF) was resuspended in the fractionation buffer, and the supernatant was aliquoted as cytosolic fraction. Lysosomal pH measurement in live cells Cells grown on a six-well plate were incubated with 30 μg ml −1 Oregon Green-514 conjugated dextran for overnight. The following day, cells were incubated in a serum-free medium for 1 h and then collected by trypsinization. Cells were resuspended in 200 μl of HBSS. The fluorescence of sample was measured at 530 nm by excitation at 440 and 490 nm at 30 s intervals for 10 min using a 96-well plate reader (Infinite M200, Tecan, USA). The average of collected values was interpolated to a pH calibration curve that was plotted by control cell aliquots in nigericin (10 μg ml −1 ) containing buffered isotonic solutions (pH 3–7). In vitro lysosome acidification assay This assay was performed as previously described [11] with a few modifications. Cells were grown in a culture medium supplemented with 30 μg ml −1 Oregon Green-514 conjugated dextran (Molecular Probes, USA) for overnight, and then incubated in a serum-free medium for 2 h followed by 1 μM carbonyl cyanide 4-(trifluoromethoxy) phenylhydrazone (FCCP) treatment for 15 min. Lysosome fraction was prepared in the presence of 1 μM FCCP. The LEF was then resuspended in 180 μl of fractionation buffer without FCCP and transferred to a black 96-well plate. The baseline fluorescence of sample was first measured at 530 nm by excitation at 440 and 490 nm at 30 s intervals for 5 min using a 96-well plate reader (Infinite M200, Tecan). The acidification of LEF by v-ATPase was initiated by adding 5 mM ATP and 5 mM MgCl 2 , and the fluorescence measurement was resumed for 30 min. To verify the specificity of assay, 100 nM bafilomycin-A 1 (Cayman Chemicals, USA) was directly added to the resuspended LEF. Generation of stable MEF cell lines To generate the TFEB-GFP expressing cells, pEGFP-N1-TFEB plasmid (Addgene, cat. no. 38119) was sub-cloned into a retroviral vector (pMxs-IRES-Puro). Recombinant retroviruses were made by transfecting the retroviral vectors into packaging cells, and then MEFs were infected with the recombinant retroviruses. Infected cells were selected using puromycin (4 μg ml −1 ). The GFP-TFEB S142A plasmid was constructed by a quick-change mutagenesis method using the above retroviral plasmid as template. Myc-tagged human Rheb cDNA was PCR amplified and sub-cloned into pMxs-IRES-Puro vector. The constitutively active mutant (Rheb S16H ) was constructed by a quick-change mutagenesis method. qRT–PCR analysis Total RNA was prepared from tissues or MEFs using either Trizol solution (Invitrogen) or RNeasy Plus mini kit (Qiagen, Germany), and 200 ng of total RNA was reverse transcribed using iScript cDNA Synthesis kit (Bio-Rad, USA). cDNA (10 ng) mix was added to KAPA SYBR FAST Master Mix (KAPA Biosystems, USA) with specific primer sets (0.5 μM; Supplementary Table 1 ), and the PCR was performed using ABI 7300. All C t values were normalized with hypoxanthine-guanine phosphoribosyltransferase (HPRT) and the relative expression level was determined using the 2 −Δ C t method (Δ C t sample = C t sample – C t geomean of housekeeping genes ). Immunohistochemistry and histological analysis Surgically removed tissues were immediately fixed in 4% paraformaldehyde (Electron Microscopy Sciences, USA)+PBS solution for overnight followed by paraffin embedding. For immunohistochemistry, deparaffinized tissue sections were rehydrated and then microwaved for 5 min in 10 mM sodium citrate buffer (pH 6.0) for the epitope retrieval. After quenching of endogenous peroxidase activity and blocking procedures, the tissue sections were incubated with primary antibodies for overnight at 4 °C. For all rabbit IgG primary antibodies (listed in Supplementary Table 2 ), the immunostaining was performed using a Vectastain elite ABC kit and a DAB peroxidase substrate kit (Vector Laboratories, USA) according to the manufacturer’s instruction. Otherwise, horseradish peroxidase-conjugated secondary antibodies were used for the staining. The antibody list can be found in the supplementary information . Other histological stains such as haematoxylin and eosin, Masson’s trichrome and Peridodic Schiff staining were performed by the University of California-San Diego (UCSD) histology core. Immunoblot analysis Snap-frozen tissues were homogenized in a cold tissue lysis buffer (1% SDS, 1% NP-40, 50 mM NaF, 2 mM EDTA, 1 mM Na 3 VO 4 , protease inhibitor cocktail tablet (Roche, Germany), 100 mM NaCl and 10 mM Tris-HCl, pH 7.5) followed by centrifugation at 13,000 g for 10 min at 4 °C to remove undissolved materials. Protein concentration was determined using detergent compatible protein assay reagents (Bio-Rad) and equal amount of total protein was used for SDS–PAGE. After the resolved proteins were transferred on polyvinylidene difluoride (PVDF) membrane (Millipore, USA), the membrane was incubated with primary antibody diluted in 5% bovine serum albumin (BSA)+Tris-buffered saline+tween20 (TBST) buffer for overnight at 4 °C. Antibody bound target proteins were detected with horseradish peroxidase-conjugated secondary antibodies and ECL solution. MEFs (1 × 10 5 ) were plated on a well of 12-well plate and cultured overnight in high-glucose DMEM medium (Invitrogen) supplemented with 10% fetal bovine serum (Hyclone) and penicillin (100 unit ml −1 )/streptomycin (100 mg ml −1 , Gibco, USA). For the autophagy flux induction, cells were first replenished with a fresh medium and then incubated in HBSS (Mediatech Inc., USA) for the indicated time period in the absence or in the presence of 100–200 nM bafilomycin-A 1 (Cayman Chemicals). After a rinse with PBS, cell lysates were collected in 1 × SDS sample buffer followed by SDS–PAGE. For the quantification of immunoblot data, the densitometry of scanned images was measured using the Quantity One software (Bio-Rad). The un-cropped scanned images of immunoblots can be found in the Supplementary Information ( Supplementary Fig. 6 ). Transmission electron microscopy Mice were perfused with modified Karnovsky’s fixative (2.5% glutaraldehyde and 2% paraformaldehyde in 0.15 M sodium cacodylate buffer, pH 7.4), and collected tissues were cut into small pieces followed by incubation in the fixative for overnight at 4 °C. Ultrathin sections were prepared by UCSD electron microscopy facility and examined using a JOEL 1200EX II transmission electron microscope. Glycogen measurement About 10–20 mg of snap-frozen tissue was homogenized in 200 μl deionized H 2 O followed by boiling for 5 min. The boiled homogenates were spun down at 16,000 g for 5 min, and 10 μl of the supernatant was used for the assay. The glycogen level was determined using EnzyChrom glycogen assay kit (BioAssay System, USA) as instructed by the manufacturer. Glycogen phosphorylase activity assay Snap-frozen tissues (20–80 mg) were homogenized in 200–800 μl imidazole buffer (0.5 mM DTT, 5 mM EDTA, 20 mM KF and 50 mM imidazole solution, pH 7.0). The homogenates were centrifuged at 13,000 g for 10 min at 4 °C. A quantity of 10 ml of the supernatant was added to 200 μl of reaction buffer (50 mM imidazole solution, pH 7.0, 20 mM glycogen, 20 mM K 2 HPO 4 , 0.5 mM MgCl 2 , 1 mM EDTA, 0.1 mM NADP+, 2 μM glucose 1,6-bisphosphate, 0.5 mM DTT, 0.025% BSA, 0.6 U ml −1 P -glucomutase, 1 mM 5′AMP and 1 U ml −1 glucose 6-phosphate dehydrogenase). NADPH production by the enzymatic reaction was measured at 450 nm by excitation at 350 nm (1 min intervals for 1 h). Immuno-purification of RagA proteins HEK293A cells were co-transfected with plasmids encoding Flag-RagA and RagC using PolyJet DNA In Vitro Tranfection reagent (SinaGen Lab). After 48 h of transfection, cells from two dishes (15 cm) were collected using mild lysis buffer (MLB; 10 mM Tris-HCl, pH 7.5, 2 mM EDTA, 100 mM NaCl, 1% NP-40, 50 mM NaF, 1 mM Na 3 VO 4 and protease inhibitor cocktail (Roche)). After centrifugation, the supernatants were transferred and then incubated with the anti-Flag resin (Sigma-Aldrich, USA). The resin was washed three times with MLB and elution was carried out with buffer containing 20 mM Tris, pH 7.5, 5 mM EDTA and 3 × flag-peptide. Eluted proteins were loaded onto a column (Pierce) to remove detergent followed by dialyzation in fractionation buffer. Purified protein was visualized by Coomassie blue staining and the protein concentration was determined. Sialidase A treatment Cells were plated on 12-well plate and cultured for overnight. Cells were then collected in MLB and the cell lysates were denatured using a Glyopro Enzymatic Deglycosylation Kit (Prozyme, USA). Denatured lysates were incubated with 2 μl of sialidase A at 37 °C for 3 h as instructed by the manufacturer. Echocardiography Two- to six-month-old male and female mice were anaesthetized by intraperitoneal injection of 2,2,2-tribromoethanol (Sigma-Aldrich, 300 mg kg −1 ). After shaving the chest, the animal was placed on a warm pad, and echocardiograph examination was performed by using Acuson Sequoia C256 (Siemens Medical Solutions). A 13-MHz linear ultrasound probe was used. All the measurements of LV internal diameter were taken in M-mode short axis. LVEDD was measured at the time of the apparent maximal LV diastolic dimension, whereas LV end-systolic diameter (LVESD) was measured at the time of the most anterior systolic excursion of the posterior wall. In the same positions, diastolic and systolic wall measurements were taken. LV FS expressed in percentages was calculated as follows: FS=(LVEDD−LVESD)/LVEDD × 100. Mitral inflow peak E and A wave velocities were also measured. Haemodynamic analysis Two- to six-month-old male and female mice were anaesthetized by intraperitoneal injection of 2,2,2-tribromoethanol (Sigma-Aldrich, 300 mg kg −1 ) and the right carotid artery was cannulated with a high-fidelity microtip pressure transducer catheter (1.4 Fr, Model SPR-839; Millar Instruments, Houston, TX). The catheter was advanced into the aorta to measure aortic pressure and into the LV to measure LV function and pressures. LV pressure and +d P /d t and −d P /d t (change in pressure over time) were recorded using a chart recorder (Model MT95K2; Astro-Med, West Wanwick, RI). Statistical analysis P (two-sided) values were determined by the Wilcoxon rank sum or signed rank (for paired samples) test for the comparison of two experimental groups using Mstat software (Dr Drinkwater, University of Wisconsin-Madison). For the comparison of survival curve, the Mantel–Cox (log-rank) test was used. How to cite this article: Kim, Y. C. et al. Rag GTPases are cardioprotective by regulating lysosomal function. Nat. Commun. 5:4241 doi: 10.1038/ncomms5241 (2014).